Mechanisms of carbon storage in mountainous headwater rivers Published research emphasizes rapid downstream export of terrestrial carbon from mountainous headwater rivers, but little work focuses on mechanisms that create carbon storage along these rivers, or on the volume of carbon storage. Here we estimate organic carbon stored in diverse valley types of headwater rivers in Rocky Mountain National Park, CO, USA. We show that low-gradient, broad valley bottoms with old-growth forest or active beaver colonies store the great majority of above- and below-ground carbon. These laterally unconfined valley segments constitute <25% of total river length, but store ∼ 75% of the carbon. Floodplain sediment and coarse wood dominate carbon storage. Our estimates of riverine carbon storage represent a previously undocumented but important carbon sink. Our results indicate that: not all mountainous rivers rapidly export carbon; not all valley segments are equally important in carbon storage; and historical changes in riverine complexity have likely reduced carbon storage. The amount of carbon that rivers deliver to oceans represents only about a third of the terrestrial carbon entering rivers [1] . The flux of organic carbon mobilized into rivers, however, is much greater than the river network’s capacity to stabilize the carbon via organo-mineral complexation or anoxic burial. Nearly half the organic carbon introduced into streams is rapidly metabolized or photolysed and returned to the atmosphere as CO 2 (ref. 1 ), Consequently, rates of erosion, delivery and mixing of fresh mineral surfaces with organic matter likely control watershed- to global-scale carbon sequestration fluxes [1] . Recent work emphasizes the importance of headwater rivers in this context. Headwater rivers receive the bulk of terrestrial carbon entering a river network [2] . Headwaters contribute significantly to CO 2 outgassing via microbial activity [3] , which partly reflects the geomorphic complexity of low-order streams created by spatial variations of hydraulics and substrate [4] . In temperate environments and higher latitudes, headwater rivers can also store disproportionate amounts of carbon in coarse dead wood relative to downstream portions of river networks [5] . The rate at which organic matter is delivered to headwater rivers, and the conditions that facilitate either storage or downstream export of this organic matter, thus exert important influences on watershed-scale carbon fluxes. Mountainous rivers contribute disproportionately to delivery of sediment and organic carbon to the oceans [6] , [7] , [8] . Research in the mountainous tropics demonstrates that headwater rivers respond to disturbances, such as cyclones, landslides and large floods, by rapidly exporting terrestrial carbon downstream [6] , [9] , [10] , [11] . Headwater rivers in the temperate zone and at higher latitudes, which typically have less frequent and intense disturbances than tropical rivers [12] , [13] , may not transmit organic carbon downstream as rapidly. However, little work has focused on mechanisms that contribute to creating carbon storage, or on the volume of carbon stored, along headwater rivers with less intense disturbance regimes. Watershed-scale carbon sequestration fluxes in tropical rivers may strongly reflect episodic disturbances, such as landslides and floods, whereas fluxes in rivers with less intense disturbance regimes may strongly reflect river geomorphic complexity that facilitates carbon storage. Geomorphic complexity in this context includes channel-spanning obstructions such as logjams or beaver dams that facilitate transient carbon storage and enhanced biological uptake over a few hours in a pool, as well as sequestration via sedimentation over thousands of years on a floodplain [2] , [3] , [14] , [15] , [16] . Few studies examine how geomorphic complexity of mountainous headwater rivers influences carbon dynamics, and particularly how headwater rivers with infrequent natural disturbances in the form of intense rainfall or large floods may store substantial volumes of carbon. We use field data from mountainous headwater rivers in CO, USA ( Fig. 1 ) to examine (i) distribution of carbon storage in this river network, (ii) magnitude of storage in different valley types, (iii) mechanisms facilitating storage and (iv) how human alteration of these rivers and the greater landscape has likely reduced the magnitude and future potential of carbon retention. Here, mechanisms refer to physical and biological processes such as logjams and beaver dams that increase overbank flooding and channel geomorphic complexity. We focus on headwater river networks in Rocky Mountain National Park because the park includes the largest remaining stands of old-growth forest and some of the least altered mountain streams and valley bottoms in the region. Although old-growth forests are now rare, forests in many mountainous regions historically resembled the study area in having a mosaic of differently aged stands caused by wildfire, hill slope instability and other natural disturbances. By including valley segments with old-growth and younger forest, we evaluate how loss of old-growth forest might influence carbon storage. We find that diverse valley segments have significantly different partitioning of organic carbon and significantly different total organic carbon storage. Unconfined valleys with old-growth forest have much greater carbon storage in coarse wood, and all unconfined valley segments have especially large organic carbon storage in floodplain sediment. Unconfined valley segments store ∼ 75% of total carbon within the river network, despite constituting <25% of the total river length. Extrapolating to the watershed scale, valley bottoms throughout the network represent <1% of the surface area in the watershed, but store nearly a quarter of the organic carbon in the watershed. 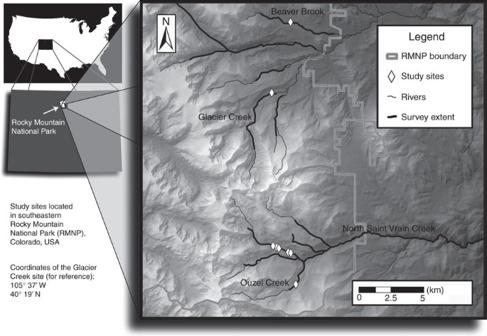Figure 1: Location map of the river networks characterized in this study. The detailed map shows the North St Vrain Creek, Glacier Creek and Beaver Brook drainages on the eastern side of Rocky Mountain National Park, CO, USA. The darker line segments within the river network indicate the length of channel mapped for different valley types. White diamonds indicate the 100-m valley segments characterized in this study. Figure 1: Location map of the river networks characterized in this study. The detailed map shows the North St Vrain Creek, Glacier Creek and Beaver Brook drainages on the eastern side of Rocky Mountain National Park, CO, USA. The darker line segments within the river network indicate the length of channel mapped for different valley types. White diamonds indicate the 100-m valley segments characterized in this study. Full size image Headwater rivers in Rocky Mountain National Park Headwater rivers of Colorado in common with rivers in other mountainous environments, have pronounced downstream variations in valley geometry [12] . 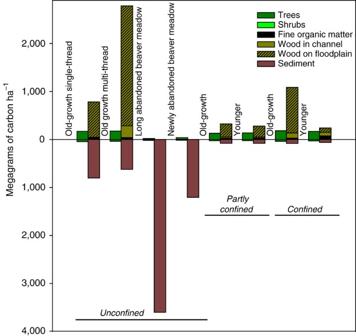Figure 2: Carbon pools (Mg per ha) of different ecosystem components within each of the eight valley types. Components of aboveground biomass are shown above thexaxis; below-ground carbon components are shownbelow thexaxis. Quantities of carbon in tree regeneration and herbaceous vegetation are too small to be visible in this figure. Spatially abrupt changes in downstream gradient and lateral confinement create valley segments 10 1 –10 3 m long that we differentiate as confined, partly confined and unconfined (Table 2) [17] . Confined segments are steep and narrow, with extensive bedrock exposure and minimal riparian vegetation. Partly confined segments have a steep bedrock wall close to one side of the channel, with a floodplain and riparian vegetation along the other side. Unconfined valley segments have a floodplain and riparian zone much wider than the channel along both sides of the valley. Unconfined valley segments can have multi-thread channels, but only if biotic drivers in the form of beaver dams or closely spaced channel-spanning logjams associated with old-growth forest are present [18] , [19] . Otherwise, single-thread channels occur. Before intensive human manipulation of rivers and adjacent forests starting in the first decades of the nineteenth century, beaver colonies and patches of old-growth forest were widespread [19] . As the occurrence of multi-thread channels depends on flow divergence caused by biotic drivers, complex multi-thread channels were likely much more abundant before beaver removal and harvest of old-growth forests. Carbon storage within individual valley segments Diverse valley segments have significantly different partitioning of organic carbon among the four reservoirs studied (floodplain sediment, coarse dead wood, fine organic matter and vegetation), and significantly different total organic carbon storage ( Fig. 2 ; Table 1 ). Unconfined valley segments with active and abandoned beaver meadows have relatively little carbon in coarse wood, but contain large volumes of carbon in floodplain sediment. Unconfined valleys with old-growth forest have much greater carbon storage in coarse wood than other valley types. In the forested reaches, vegetation carbon totals on a per area basis are similar across valley types, despite differences in disturbance history and forest age ( Fig. 2 ). Biomass carbon totals (vegetation+coarse wood+fine organic matter) are consistently higher, however, than reported for upland forest stands with similar species composition [20] . Unconfined valley segments have especially large organic carbon storage in floodplain sediment. The estimated total proportion of carbon storage in Table 1 indicates that unconfined valley segments are disproportionately important, storing ∼ 75% of total carbon within the river network, despite constituting <25% of the total river length. Figure 2: Carbon pools (Mg per ha) of different ecosystem components within each of the eight valley types. Components of aboveground biomass are shown above the x axis; below-ground carbon components are shown belo w the x axis. Quantities of carbon in tree regeneration and herbaceous vegetation are too small to be visible in this figure. Full size image Table 1 Summary of characteristics of eight representative valley segments. Full size table Carbon storage at the watershed scale We used data on ecosystem carbon stocks and export from Glacier Creek watershed ( Fig. 1 ) to estimate carbon storage and flux within North St Vrain Creek watershed, where most of our study sites are located. North St Vrain Creek watershed within Rocky Mountain National Park includes ∼ 9,000 ha, of which 65% (5,900 ha) is forested. Assuming 260 Mg C ha −1 in forested uplands [20] , and river export averaging 10 kg C ha −1 per year based on previous work [21] , [22] and our measurements of dissolved organic carbon (DOC) in North St Vrain Creek during the 2011 snowmelt runoff ( Table 2 ), we estimate 1,534 × 10 3 Mg C in forested upland portions of the watershed and river export in the range of 60–100 Mg C per year from the forested uplands. Estimates of total biomass decomposition in uplands average 1.42 Mg C ha −1 per year [20] , or 0.5% loss each year. We cannot adequately constrain the magnitude and recurrence interval of hill slope and other forest disturbances (for example, debris flows, forest blowdowns, wildfires) to develop a complete carbon balance for the watershed, but we can compare magnitudes of carbon storage in upland and riverine portions of the watershed, and use these to infer rates of carbon input to the riverine environment. Assuming that the volume of stored organic carbon that we measured per 100 m segment for each valley type is representative of that valley type, and extrapolating to the length of that valley type along the surveyed channel network within North St Vrain Creek watershed, we estimate total storage of ∼ 353,520 Mg C in valley bottoms throughout the watershed. This number is ∼ 23% of the total carbon storage estimated for forested uplands in the watershed, but underestimates carbon storage along the entire river network because our field surveys did not include small tributaries, portions of the river network above timberline ( Fig. 1 ) and associated wetlands. To put these numbers in perspective, the portion of the river network that we surveyed, which represents <1% of surface area in the watershed, stores nearly a quarter of the carbon in the watershed. Table 2 Results from DOC stream sampling. Full size table Floodplain sediment and coarse wood are the dominant reservoirs of carbon storage. This organic carbon is sourced from upstream and upslope and presumably replaced at the source site by continued soil development and forest regrowth. Radiocarbon ages on floodplain sediment are modern to depths of ∼ 20 cm, but dates on sediment from depths >30 cm reflect longer storage (ages ranging from 265±85 to 5,920±30 BP) (ref. 23 ). Large diameter dead wood requires more than a century to decay in this environment [24] . Floodplain sediment and coarse wood thus represent a potentially important and largely unrecognized form of organic carbon storage over time spans of 10 2 –10 3 years. Carbon accumulation and retention The estimates of disproportionately high-carbon storage in unconfined valley bottoms relative to uplands imply some mechanism for carbon accumulation and retention in valley bottoms. Four processes are likely to result in concentrated carbon storage along unconfined valley segments. First, dissolved and particulate organic carbon in transport within the river network is preferentially deposited along floodplains in unconfined valley segments, particularly when flow is forced out of the channel by obstructions such as logjams and beaver dams ( Fig. 3 ). This overbank flow moves slowly across the hydraulically rough floodplains, resulting in infiltration and high riparian water tables, as well as deposition and burial of particulate organic matter. Second, high riparian water tables, especially in valley segments with numerous beaver dams, result in saturated soils that limit microbial decomposition of organic matter [25] . The unconfined valley segments maintained high water tables and samples from particularly wet sites contained up to 17% total organic carbon. The organic horizons of upland soils in this region typically contain <10% total organic carbon [26] . Third, as reflected in Fig. 2 , coarse wood in the channels and floodplain constitutes a substantial carbon reservoir. Coarse wood in transport within the river network is preferentially deposited along channels in wider, lower-gradient valley segments because of reduced transport capacity relative to the steep, narrow valley segments [27] . In unconfined valley segments with old-growth riparian forests, most wood is retained on site as trees die and fall. Because of the wide riparian area, high stem density and larger diameter trees, this substantial pool of stored carbon continues to accumulate over time. Large diameter trees decay very slowly: complete decay for the dominant conifer species in this environment requires 300–900 years [28] . Fourth, in unconfined valley segments in the subalpine forest zone at higher elevations of the study area, annual peak flows result from snowmelt. These peak flows can inundate the valley bottom, but do not generate sufficient hydraulic force to substantially erode the floodplain surface. Erosion of floodplain sediments results instead from bank erosion associated with more gradual lateral movement of channels. This results in longer residence time of floodplain sediments, as reflected in the presence of trees >300 years old growing next to the channel. In contrast, valley segments at lower elevations may experience episodic erosion that completely strips the floodplain of stored sediment and organic matter. This type of large-scale floodplain erosion can occur where convective rainfall can generate flash floods with large peak discharge [29] . Together, these four processes contribute to concentrated storage and persistence of organic carbon along unconfined valley segments. 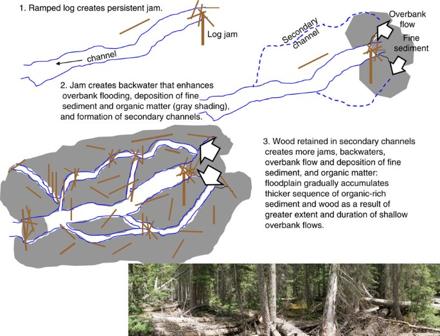Figure 3: Schematic illustration of the feedback effects of a channel-spanning logjam on carbon storage. In the absence of a sufficient number and size of logs to form persistent jams and overbank flooding, a single-thread channel is maintained with high transport capacity for wood, fine sediment and organic matter, and limited deposition across the floodplain. Along unconfined stream segments with old-growth riparian forests, characterized by high stem densities and large diameter trees, large volumes of wood enter the stream and create channel-spanning logjams at frequent intervals down the channel. Each of these obstructions creates backwater and sedimentation upstream, and facilitates overbank flow across the floodplain. Overbank flow enhances the deposition of dissolved and particulate organic matter being transported by stream flow. Also, shallow overbank flows move slowly across the topographically rough floodplain with limited erosional capability, so on-site organic matter is retained and incorporated into litter and duff layers on the forest floor (fine organic matter inFig. 2). Fallen wood from the riparian forest also remains in place, rather than being transported downstream, further contributing to carbon storage on the floodplain, as reflected in the photo at the bottom of the illustration. This photo is a portion of the valley bottom at the unconfined, old-growth, multi-thread channel valley segment characterized for this study. Note the abundant wood on the forest floor. In all cases, flow is from upper right toward lower left. Figure 3: Schematic illustration of the feedback effects of a channel-spanning logjam on carbon storage. In the absence of a sufficient number and size of logs to form persistent jams and overbank flooding, a single-thread channel is maintained with high transport capacity for wood, fine sediment and organic matter, and limited deposition across the floodplain. Along unconfined stream segments with old-growth riparian forests, characterized by high stem densities and large diameter trees, large volumes of wood enter the stream and create channel-spanning logjams at frequent intervals down the channel. Each of these obstructions creates backwater and sedimentation upstream, and facilitates overbank flow across the floodplain. Overbank flow enhances the deposition of dissolved and particulate organic matter being transported by stream flow. Also, shallow overbank flows move slowly across the topographically rough floodplain with limited erosional capability, so on-site organic matter is retained and incorporated into litter and duff layers on the forest floor (fine organic matter in Fig. 2 ). Fallen wood from the riparian forest also remains in place, rather than being transported downstream, further contributing to carbon storage on the floodplain, as reflected in the photo at the bottom of the illustration. This photo is a portion of the valley bottom at the unconfined, old-growth, multi-thread channel valley segment characterized for this study. Note the abundant wood on the forest floor. In all cases, flow is from upper right toward lower left. Full size image For purposes of comparison, uplands in this region are estimated to have net primary production of 2.8 Mg C ha −1 per year and decomposition of 1.42 Mg C ha −1 per year, resulting in net carbon balance of 1.38 Mg C ha −1 per year [20] . Carbon pools and fluxes are remarkably consistent across diverse forested subalpine sites. Carbon pools increase with stand age and time since forest disturbance, although detrital carbon stored in the upland forest floor is more variable, partly as a function of the history of wildfire and surface erosion [20] . Floodplains with old-growth forest are likely to have the greatest carbon pools in the region and low disturbance and surface erosion. If we use the regional estimate of 1.38 Mg C ha −1 per year net carbon balance and an average value of 2,350 Mg C ha −1 in unconfined valley segments, this suggests ∼ 1,700 years to accumulate measured carbon stocks in unconfined valley segments. This is likely an overestimate of time required to accumulate carbon because of the mechanisms described above that concentrate carbon storage in unconfined valley bottoms. However, 1,700 years is not unreasonable given the range of radiocarbon ages of floodplain sediment and organic matter at the study sites. The first-order approximations of carbon storage in floodplain sediment and coarse wood presented here have at least three important implications. First, valley segments differ markedly with respect to carbon storage. Greater valley-bottom area, greater floodplain sediment depth and large amounts of down coarse wood in old-growth stands create the greatest storage of organic carbon in unconfined valley segments of the study area. Within these segments, old-growth forest or beavers are critical to retention of biomass carbon and carbon-rich floodplain sediment ( Fig. 3 ). The large trees of old-growth stands eventually become stored carbon in dead wood and, if recruited to the channel, facilitate formation of channel-spanning logjams that create backwater depositional areas and enhance overbank flow and floodplain deposition and organic carbon retention [17] . Beaver dams similarly enhance overbank flow, floodplain deposition and organic matter retention, and maintain high water tables that support dense stands of willow ( Salix spp.) and other riparian shrubs [30] , [31] , [32] . The unequal distribution throughout the river network of carbon stored in floodplain sediment and coarse wood suggests that resource management designed to facilitate carbon storage can be most effectively focused on the relatively small proportion of channel segments with unconfined valleys. The second implication of our results involves historical changes in mountain headwater rivers that have altered channel form and process and carbon dynamics. In the absence of logjams and beaver dams, valley geometry does not change, but channel-floodplain interactions that facilitate overbank deposition and floodplain carbon storage change. Along reaches dominated by younger riparian forest with small diameter trees, jams that can force overbank flow are more widely spaced and transient [17] , [18] . Much less carbon is stored in dead wood than in reaches with older forests. In the absence of active beaver colonies, beaver dams decay and break apart. In abandoned beaver meadows, riparian water tables drop and vegetation becomes less productive. In both scenarios, depth, extent and duration of overbank flooding decrease, less organic matter is deposited on the floodplain and stored floodplain carbon can be oxidized or eroded [31] . Consequently, the amount of carbon stored in living and dead biomass declines. The net effect of diverse resource uses, including beaver trapping, timber harvest, log floating and flow regulation in western North America and other mountainous regions around the world [33] , [34] , has been reduction in the extent of old-growth forest and, in North America and Eurasia, the abundance and distribution of beavers ( Castor canadensis and Castor fiber , respectively) [35] . The loss of these biotic drivers, along with channelization of multi-thread channels into single channels, levees that reduce or eliminate overbank flooding and removal of instream wood, has substantially reduced the physical complexity of mountainous headwater rivers [16] . Loss of geomorphic complexity and channel-floodplain connectivity equates to reduced organic carbon storage. Headwater rivers become ‘leaky’, rapidly transporting sediment and organic matter downstream, rather than retaining these materials along valley bottoms [18] . This reduces headwater river ecosystem productivity and can create water-quality problems for downstream drinking water supplies. A critical consideration with respect to historical changes is that many headwater rivers have lost geomorphic complexity during recent centuries [34] . Alterations associated with land use and manipulation of rivers have simplified channel and riparian features along many headwater river networks [36] . However, the implications for carbon storage have not been previously considered. The mechanisms and residence time of floodplain organic carbon storage described here are likely similar in temperate or high-latitude headwater rivers. Disturbance regimes in mountainous watersheds are characterized by fire, wind and subsequent blowdown, and forest insect infestations that are more likely to contribute to changes in carbon storage, distribution and decomposition than rapid carbon export. The third implication of our work is that not all mountainous headwater rivers rapidly export carbon. Relative to tropical mountainous headwater rivers with large carbon fluxes to the ocean [6] , [8] , [9] , [10] , [11] , the headwater rivers described here respond differently to carbon delivery from upland sources and can store substantial quantities of carbon. Global compilations indicate that temperate forest watersheds typically have lower organic carbon export than other environments, including boreal forest, wetlands and tropical forests [8] , [21] . Work in Glacier Creek, CO indicates that subalpine forests in our study region have low production relative to other temperate coniferous forests [37] , as well as low rates of riverine carbon export [22] . Estimates of carbon storage in headwater floodplain sediment, however, are largely undocumented. One recently published estimate of floodplain carbon storage in the Rhine River catchment, for example, excludes mountainous portions of the catchment [38] . An exception is recent research on floodplain wetlands buried under historic milldam sediments along headwater streams in the eastern United States: the wetland sediments contain 250–1,350 Mg C ha −1 (ref. 39 ). By comparison, our unconfined valley segments contain 60–1,000 Mg C ha −1 in sediment and 500–3,600 Mg C ha −1 total. Although individual headwater floodplains are much narrower and shallower than the extensive floodplains that characterize downstream portions of large river networks, the cumulative length of the many small tributaries in a river network implies that organic carbon storage along these smaller rivers can be important. Further study of mechanisms and patterns of carbon storage in diverse geographic settings is needed to determine regional differences and the relative abundance of headwater rivers characterized by large downstream carbon fluxes [6] , [8] , [9] , [10] , [11] versus headwater rivers characterized by the storage mechanisms described here. However, widespread reduction of geomorphic complexity along headwater channels likely has long-term and cumulative global effects on the carbon cycle. Although old-growth forests and beaver colonies have become scarce, our findings of concentrated organic carbon storage along valley segments regulated by these biotic drivers provide further incentive to reduce beaver removal and deforestation. Our research also implies that anticipated effects of a warming climate (for example, increased frequency and intensity of wildfire in the Rocky Mountains) that limit the establishment or continuation of old-growth forest may reduce carbon storage along headwater river corridors. Patterns observed in this river network likely apply to those in other temperate mountainous headwaters, with broad consequences for understanding global carbon sequestration, managing biotic–river interactions and planning for sustainable freshwater resources. Study area Geology, geomorphic history, climate and upland vegetation are consistent across the valley segments studied here, which are underlain by Precambrian-age crystalline rocks that weather relatively slowly in the semiarid environment. Pleistocene valley glaciers extended to elevations below the 2,900–2,500 m range of the study sites, which today are covered in subalpine forest of lodgepole pine ( Pinus contorta ), spruce ( Picea spp.) and fir ( Abies spp.). We examined eight types of valley-bottom segments, differentiated on lateral confinement, stand age of the riparian forest and status of beaver meadows ( Table 1 ). Old-growth forest is ≥200 years old [24] . Beaver meadows are wet meadows with beaver dams and willow communities [35] , [40] , [41] , [42] . Abandonment by beavers results in breached dams, decreased overbank flooding, lowered local water table and a progressive shift from meadow to more xeric upland vegetation [25] , [36] , [37] . For each valley type, we chose a representative 100-m valley length and quantified carbon storage in four reservoirs: floodplain fine sediment, coarse dead wood, fine organic matter and floodplain vegetation. Organic carbon in floodplain sediment Thickness of floodplain sediment finer than cobble size was measured at 10 min interval along 11 transects perpendicular to the valley long axis and spaced 10 m apart downstream. At each point, we measured thickness of fine sediment overlying cobbles or boulders. Total volume of floodplain fine sediment was estimated for each reach using triangular irregular networks constructed in ArcMap. This procedure interpolates the thickness of sediment wedges between measured depths across reach grids. Numerous samples of the floodplain fine sediment were analysed for bulk organic carbon content and bulk density. Sediment samples were analysed at the Colorado State University Soil Testing Lab for total carbon with a LECO TruSpec CN furnace [43] . Each sample was then analysed for CO 3 -C by treating the sample with 0.4 N HCl and measuring the CO 2 loss gravimetrically [44] . Total organic carbon was calculated as total carbon-CO 3 -C. Total organic carbon values varied among the ∼ 10 samples collected for each site from <1% to >17%. We averaged percent bulk carbon content for each type of valley segment. These averages, which are 10–14%, are higher than upland forest soils in the region, which average 7.3% organic carbon in the mineral soil and range from 1.9 to 25.9% (ref. 26 ). Higher organic carbon values in floodplain sediments appear reasonable in view of the inputs of fine organic matter during overbank floods and high water tables in the valley bottoms relative to uplands. We estimated an average bulk density of 1.8 g cm −3 for floodplain sediment in beaver meadows rich in silt and clay, and 1.5 g cm 3 for other floodplain sediment. We used radiocarbon samples from wood and charcoal buried in floodplain sediments to develop some insight into residence times of carbon stored in these sediments. We dated 16 samples from the long abandoned beaver meadow, 3 samples from the newly abandoned beaver meadow and 3 samples from unconfined multi-thread channel valley segments. These samples are not sufficient in number to provide a detailed chronology or average rate of floodplain aggradation, but are instead used to estimate the residence time of carbon in this depositional environment within an order of magnitude. Organic carbon in dead wood All coarse dead wood >10 cm in diameter and 1 m in length on the ground in the active channel and across the valley bottom was measured. Length and diameter of each wood piece were used to calculate piece volume, approximating the piece as a cylinder. Total wood volume was summed for each valley segment in cubic metres. We assumed an average density of 400 kg m −3 (ref. 45 ), and a carbon content of half of the wood by weight. Organic carbon in floodplain vegetation Floodplain vegetation includes live and dead standing trees, conifer regeneration in the understory, shrubs, herbaceous plants and roots of live plants. For each reach, biomass of above-ground (AG) ecosystem components was estimated by sampling within equally spaced belt transects (5 m wide) perpendicular to the channel on both sides of the stream. Width of the riparian areas varied considerably across valley types: number and length of belt transects were determined for each reach to sample at least 20% of reach area. Diameter at breast height of live and dead trees (≥5 cm) was recorded by species and AG biomass calculated using published allometric equations [46] . For live trees, below-ground (BG) biomass was estimated as 20% of AG biomass [46] . BG willow biomass was estimated as equal to AG. For saplings (diameter at breast height<5 cm), seedlings (<0.5 m tall) and individual willows, plants over a representative height range were harvested, dried and weighed, and equations for calculating biomass were developed by regressing dry weights against measured plant heights. Biomass of trees, saplings and willows were converted to C content using a multiplication factor of 0.48 (ref. 47 ). Percent cover of shrub (<0.5 m tall) and herbaceous species was estimated in 0.25 m 2 quadrats along the centre line of each belt transect (5–15 quadrats per transect, depending on reach area). Vegetation within a subsample of the quadrats was harvested, dried, weighed to obtain biomass weights and analysed for C content using a LECO CHN analyser. Biomass of seedlings, shrubs and herbaceous plants were converted to C content using multiplication factors ranging from 0.42 to 0.52, depending on the biomass component. Organic carbon in litter and duff Fine organic matter is (i) litter, the top layer of the forest floor, slightly decomposed organic material that is mostly identifiable and easily removed from the surface and (ii) duff, moderately to highly decomposed organic material beneath the litter and above the mineral soil. These layers were sampled in quadrats along transect centre lines, dried, weighed and subsampled for carbon content. Biomass was converted to C content using multiplication factors ranging from 0.38 to 0.52. For each reach, total vegetation C was estimated by summing AG and BG biomass C pools and fine organic matter C pools. Watershed carbon storage As a first-order approximation, we calculated total watershed-scale carbon storage by multiplying measured carbon in each of the four reservoir types in the 100-m-long valley segment by total length of that segment type present in the river network of North St Vrain Creek within the boundary of Rocky Mountain National Park. We mapped the distribution of valley segment types within this river network by walking the mainstem and major tributaries, using a handheld global positioning unit to note the upstream and downstream boundary of each valley segment. We summed the cumulative total length of each valley segment type and calculated the proportion of total valley-bottom carbon storage associated with that type. Riverine carbon export We used two approaches to estimate riverine export of carbon. The first is based on published values averaging 10 kg C ha −1 per year for watersheds of ∼ 1,200–6,700 km 2 in the South Platte River basin of CO, which includes our study area [21] and measured DOC values at Glacier Creek watershed immediately to the north of our study area, where DOC concentrations are <1 mg C per l by late July and fall at the lower range for temperate surface waters [22] . At 59 km 2 of forested watershed in North St Vrain Creek, these values result in estimates of 59 Mg C per year exported. The second approach was based on water samples collected for DOC analysis at three time intervals during the snowmelt runoff season of 2011. This year had an unusually sustained peak snowmelt flow, with higher flows lasting through June and July before returning to base flow in August. We collected samples on 23 June 2011 (discharge 9.8 m 3 s −1 ), 20 July 2011 (discharge 10.4 m 3 s −1 ) and 23 August 2011 (discharge 2.6 m 3 s −1 ). On each of these dates, we collected ten samples along the length of North St Vrain Creek, from <1 km below Thunder Lake at the headwaters, to the eastern boundary of Rocky Mountain National Park, ∼ 20 river km downstream. All samples were filtered through a 47-mm glass fibre (GF/F) filter (0.7-mm nominal cutoff) using a hand pump at low pressure (100 mm Hg) and maintained frozen until analysis. DOC was analysed using a Shimadzu T5000. We used the average of the ten samples on each date to represent a monthly average for the watershed and assumed that values during base flow are <1 mg C per l based on the August values and research in Glacier Creek [22] . We used these data with monthly mean discharge for the North St Vrain Creek at Allenspark stream gage (USGS 6721500) over the period of record (1925–present) to calculate approximate monthly and annual export of DOC from the watershed. These values result in an estimated 103 Mg C per year of riverine export. How to cite this article: Wohl, E. et al. Mechanisms of carbon storage in mountainous headwater rivers. Nat. Commun. 3:1263 doi: 10.1038/ncomms2274 (2012).